Force-dependent conformational switch of α-catenin controls vinculin binding Force sensing at cadherin-mediated adhesions is critical for their proper function. α-Catenin, which links cadherins to actomyosin, has a crucial role in this mechanosensing process. It has been hypothesized that force promotes vinculin binding, although this has never been demonstrated. X-ray structure further suggests that α-catenin adopts a stable auto-inhibitory conformation that makes the vinculin-binding site inaccessible. Here, by stretching single α-catenin molecules using magnetic tweezers, we show that the subdomains M I vinculin-binding domain (VBD) to M III unfold in three characteristic steps: a reversible step at ~5 pN and two non-equilibrium steps at 10–15 pN. 5 pN unfolding forces trigger vinculin binding to the M I domain in a 1:1 ratio with nanomolar affinity, preventing M I domain refolding after force is released. Our findings demonstrate that physiologically relevant forces reversibly unfurl α-catenin, activating vinculin binding, which then stabilizes α-catenin in its open conformation, transforming force into a sustainable biochemical signal. Cell–matrix and cell–cell adhesions are required in morphogenesis during embryogenesis, tissue development during fetal life, as well as tissue maintenance during adulthood [1] . In addition to mere cell membrane adhesion, fine-tuning of transmission of mechanical load from cell to extracellular matrix (ECM) and cell to cell is also essential to these processes [2] , [3] . The molecular mechanisms underlying cell–ECM mechanosensing processes have been partly unraveled. Although cell–ECM mechanotransduction may rely on more global adaptation of the actomyosin viscoelastic networks [4] and activation of mechanosensitive channels [5] , pioneering works have demonstrated the existence of integrin-associated cytoplasmic proteins with buried sites of phosphorylation such as p130Cas [6] , and of protein–protein interactions such as talin [7] , [8] that are unmasked upon myosin II-dependent stretching. The tension-dependent conformation switch of these proteins may thus initiate the force-dependent building of adaptor complexes linking cell–matrix adhesions to the tension-generating actomyosin network. By analogy, cadherin-associated adhesion complexes might have an essential role in transducing forces at cell–cell junctions [9] , [10] . These complexes are tension adaptive, actin-cytoskeleton-associated structures, responsive to both external load and tensile force produced by intracellular myosin motors [11] , [12] . The mechanism of mechanosensing at cell–cell contacts has only been very recently investigated [13] , [14] , and α-catenin appears as a central component of the force transmission pathway. The αE isoform of α-catenin is expressed ubiquitously in early embryonic cells, and then restricted to epithelia. Its deletion is associated with impaired cadherin-mediated adhesion [15] , [16] , tissue growth, and homeostasis [17] , [18] , [19] . It has been recently hypothesized that αE-catenin may act as a mechanotransducer in the pathway that converts mechanical strain on cadherin adhesions into a cue for junction strengthening [11] . Because vinculin accumulates at mature cell–cell junctions upon actomyosin generated tension [11] , [20] , [21] , [22] and binds αE-catenin [23] , [24] , [25] , it has been proposed that α-catenin functions in concert with vinculin. Further analysis of cadherin adhesion strengthening by cell doublet force separation measurement indicates that α-catenin, vinculin and their direct interaction are required for tension-dependent intercellular junction strengthening [26] . These proteins appear as key candidates for mechanotransduction at cell–cell junctions. Vinculin is a cytoplasmic actin-binding protein enriched in both focal adhesions and adherens junctions, essential for embryonic development [27] . At focal adhesions, vinculin has a critical function in linking integrins to F-actin. Vinculin is a compact globular protein composed of successive four α-helix bundles. Five of these α-helix bundles constitute the vinculin head binding to various partners such as talin, whereas the C-terminal constitutes the vinculin tail binding to F-actin. In the cytosol, vinculin is under an inactive head to tail conformation presenting only week affinity for actin. In contrast, vinculin captured at focal adhesions by force-dependent activated talin is stabilized under an open conformation characterized by head to tail dissociation, stabilized by binding of the head to talin and high affinity binding of the tail to F-actin [28] . α-Catenin is a complex protein with strong homology with the vinculin head domain, sharing a λ-shape arrangement of α-helix bundles [29] . At cell–cell junctions, β-catenin directly binds to the N-terminus of α-catenin [30] , [31] and to the intracellular tail of cadherins [32] , [33] , forming the cadherin/β/α-catenin complex. α-Catenin possesses a domain of homodimerization and dimerizes in solution ( Fig. 1a : DD domain); however, this domain overlaps with a N-terminal β-catenin-binding domain, and homodimerization of α-catenin is inhibited by β-catenin binding [29] , [34] . The C-terminus of α-catenin contains an F-actin-binding site [25] , [35] , which associates the tertiary cadherin/β-catenin/α-catenin complex to the actin filaments [36] . Although direct binding has not been observed between the purified components of this complex in solution [37] , it is still acknowledged that α-catenin dynamically links the complex to F-actin directly, indirectly or both, allowing force transduction and strengthening of adhesions [13] , [26] , [38] . α-Catenin binds to other actin-binding proteins, such as vinculin [18] , [24] , [25] , [39] , ZO-1 (refs 25 , 40 ), afadin [41] and formin-1 (ref. 42) [42] , through sites distributed in the central part of the molecule. The actin-binding domain of α-catenin located at the C-terminus of the molecule ( Fig. 1a : FABD domain) appears to bind to the side of actin filaments, inducing conformational changes of individual filaments and preventing the binding of the branching complex Arp2/3 and the severing protein cofilin [43] . Thus, α-catenin binding to actin may favour assembly of unbranched filaments that are more protected from severing than dynamic, branched filament arrays [44] . 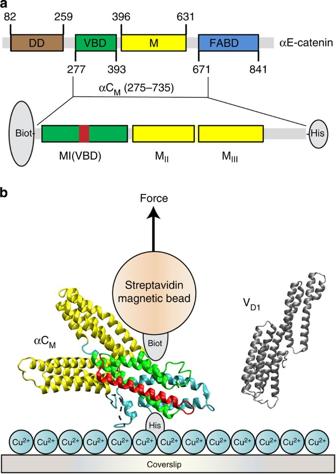Figure 1: Domain map and experimental setup. (a) Domain mapping of full-length and sub-domains of mouse αE-catenin. αE-catenin consists of an N-terminal dimerization domain (DD), followed by vinculin-binding domain (VBD; also referred to the MIdomain). Interaction between VBD and two other modulation domains (MII-MIII) is suggested to inhibit vinculin binding. αE-catenin contains a C-terminal F-actin-binding domain (FABD) that binds to F-actin and transmits mechanical forces generated by actomyosin contraction. The αCMconstruct (residues 275–735) is enclosed in the top bracket. (b) Schematics of experimental setup. A single αCMmolecule is tethered between a cover glass surface and a paramagnetic bead through NTA-His tag and streptavidin-biotin linkages, respectively. The modulatory MI(VBD) domain is shown in green, MIIand MIIIdomains in yellow. The vinculin-binding helix is marked in red. The VD1molecule, which is also a helix bundle, is shown in silver. Force was applied to the paramagnetic bead using a pair of permanent magnets. αCMconstructs were stretched in the absence or in the presence of VD1of various concentrations. The model of αCMis adopted from PDB structure 4IGG. Figure 1: Domain map and experimental setup. ( a ) Domain mapping of full-length and sub-domains of mouse αE-catenin. αE-catenin consists of an N-terminal dimerization domain (DD), followed by vinculin-binding domain (VBD; also referred to the M I domain). Interaction between VBD and two other modulation domains (M II -M III ) is suggested to inhibit vinculin binding. αE-catenin contains a C-terminal F-actin-binding domain (FABD) that binds to F-actin and transmits mechanical forces generated by actomyosin contraction. The αC M construct (residues 275–735) is enclosed in the top bracket. ( b ) Schematics of experimental setup. A single αC M molecule is tethered between a cover glass surface and a paramagnetic bead through NTA-His tag and streptavidin-biotin linkages, respectively. The modulatory M I (VBD) domain is shown in green, M II and M III domains in yellow. The vinculin-binding helix is marked in red. The V D1 molecule, which is also a helix bundle, is shown in silver. Force was applied to the paramagnetic bead using a pair of permanent magnets. αC M constructs were stretched in the absence or in the presence of V D1 of various concentrations. The model of αC M is adopted from PDB structure 4IGG. Full size image The α-catenin central domain (αC M , Fig. 1a : VBD+M domains) is an adhesion modulation domain [25] , [45] , composed of a vinculin-binding domain M I or VBD [23] , [46] , followed by the so-called modulation domains M II and M III (ref. 47 ). Biochemical and structural data suggest that the vinculin helix bundle (V D1 ) forming the vinculin head binds to a single vinculin-binding α-helix (residues 305–355) within the α-catenin VBD domain [39] , [46] . Structural data further indicate that α-catenin can adopt an auto-inhibitory conformation [48] whereby the VBD domain is interacting with both M II and M III helix bundles, thus preventing accessibility of the vinculin-binding domain. Vinculin may only bind to α-catenin when the VBD-M II -M III helix bundles are in an open conformation [46] , [47] , [48] . Altogether, these data suggest that α-catenin may unfurl in a tension-dependent manner, allowing the recruitment of vinculin, and further strengthening of the cadherin complex/F-actin linkage. This pathway may be responsible for the mechanosensitive maturation of intercellular junctions. However, crucial experiments are lacking in support of this hypothesis. No direct evidence demonstrates the force-dependent unfurling exposing the VBD α-helix and the binding of α-catenin to vinculin under force. To investigate the role of α-catenin in force transduction, we use single-molecule assays that allow us to obtain direct experimental evidence that physiological-range forces regulate α-catenin conformation and α-catenin–vinculin interaction. Thus, we provide here a molecular mechanism by which forces are locally transformed into biochemical signal at cadherin-mediated adhesions, which has significant implications for adherens junction assembly and regulation. αC M unfolds in three characteristic steps under force To experimentally test the hypothesis that the modulation domain of αE-catenin (αC M ) containing the VBD-M II -M III helix bundles can unfurl upon application of physiological-range forces [39] , we first investigated the force response of αC M domain of mouse αE-catenin (275–735), produced with a biotin tag at the N -terminal and a 6-His tag at the C-terminal ( Fig. 1a ), thanks to a stable high-force magnetic tweezers instrument [49] , [50] , [51] . For this set of experiments, we specifically tethered single αC M molecules between an NTA-Cu 2+ functionalized coverslip and a streptavidin-coated paramagnetic bead and subjected the tethered molecules to forces exerted by a pair of permanent magnets ( Fig. 1b ). We recorded the extension change of the αC M molecule based on the diffraction pattern of the bead at a sampling rate of 200 Hz with nanometer resolution [49] . To obtain a mechanical characterization of the molecule, single αC M tethers were subjected to force scanning cycles. In each cycle, force was increased at a constant loading rate of 4 pN s −1 from ~1 pN to ~40 pN, which was followed with a force-decrease step, reducing force exponentially with time back to <1 pN that minimizes duration of the tether being held at large forces ( Fig. 2a ). The chosen loading rate of 4 pN s −1 is within a physiologically relevant range, as recently estimated for integrin stretching during cell retraction [52] . During the force-increase step, we identified unfolding events by sudden increases in the extension of the αC M tether, whereas we also identified refolding events during the force-decrease step by sudden decreases in the extension. To allow refolding of the αC M molecule following the force-decrease step, we held the αC M tether at<1 pN for 1 min. During this period of time, the refolding of αC M appeared taking place with a >90% probability ( Supplementary Fig. 1a ). The unfolding and refolding force-responses that we observed indicate that αC M behaves like a nonlinear spring, which may be important for its potential in vivo function as a mechanosensor. 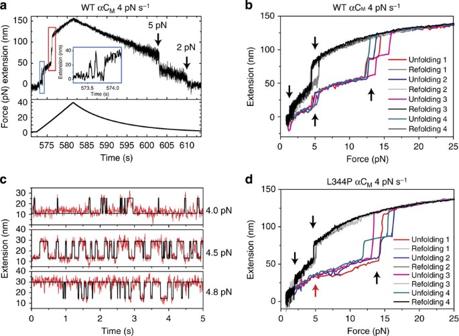Figure 2:Force response of αCM. (a) Extension change of αCMrecorded at 200 Hz in a typical force cycle experiment. During the stretch phase (force-increase) at a loading rate of 4 pN s−1, an unfolding step was observed at ~5 pN (blue box), and two additional ones occurred at higher forces (~15 pN; red box). Two refolding events, one at ~5 pN with>20 nm and another at ~2 pN with >10 nm, were observed during relaxation (force-decrease). The inset shows that the extension at ~5 pN is reversible. (b) Four force-extension curves recorded in four sequential stretch-relax cycles. The stretch curves are indicated in colour, whereas the relax curves are indicated in grey scale. Unfolding steps are marked by up arrows and refolding steps are marked by down arrows. Data inbare smoothed using 0.05-s time intervals. (c) Stepwise extension fluctuation at constant forces. Raw data are shown in red, and the black lines are fitted states using Hidden Markov method (Methods: ‘Determination of transition rates at constant forces’). (d) Typical force-extension curves obtained from four force cycles for L344P αCMmutant on a single tether. The red up arrow marks the missing ~5 pN unfolding step. Figure 2: Force response of αC M . ( a ) Extension change of αC M recorded at 200 Hz in a typical force cycle experiment. During the stretch phase (force-increase) at a loading rate of 4 pN s −1 , an unfolding step was observed at ~5 pN (blue box), and two additional ones occurred at higher forces (~15 pN; red box). Two refolding events, one at ~5 pN with>20 nm and another at ~2 pN with >10 nm, were observed during relaxation (force-decrease). The inset shows that the extension at ~5 pN is reversible. ( b ) Four force-extension curves recorded in four sequential stretch-relax cycles. The stretch curves are indicated in colour, whereas the relax curves are indicated in grey scale. Unfolding steps are marked by up arrows and refolding steps are marked by down arrows. Data in b are smoothed using 0.05-s time intervals. ( c ) Stepwise extension fluctuation at constant forces. Raw data are shown in red, and the black lines are fitted states using Hidden Markov method (Methods: ‘Determination of transition rates at constant forces’). ( d ) Typical force-extension curves obtained from four force cycles for L344P αC M mutant on a single tether. The red up arrow marks the missing ~5 pN unfolding step. Full size image In a typical force-increase scan, we found that the αC M unfolded in three characteristic steps ( Fig. 2a ). Because both extension and force at any time were known, the time traces of extension and force could be converted into force-extension curves ( Fig. 2b ). Representative unfolding and refolding force-extension curves obtained during successive force cycles on a single αC M tether shows remarkable reproducibility ( Fig. 2b ). We confirmed this reproducibility on multiple (>10) independent αC M molecules ( Supplementary Fig. 1b for another example). At a constant loading rate of 4 pN s −1 , the first step occurred at 5.2±0.7 pN (mean±s.d.) and involved a reversible extension change of 16.3±4 nm (mean±s.d.) between two conformational states, which can be understood by unfolding the bundled α-helices in the VBD domain into a linear chain of extended α-helices as discussed in the Discussion section. The inset in Fig. 2a clearly shows that the extension of the tether fluctuates at forces ~5 pN indicating that the transition of the corresponding domain is near equilibrium when the αC M tether is subjected to this force magnitude. The two higher force steps were overlapping at about 12.5±2.0 pN and had similar step sizes of 23.3±6.6 nm corresponding to 105±30 residues. These unfolding sizes fit the domain sizes of αC M (VBD: 277–393, M II -M III : 396–631, Fig. 1a ) [25] , [45] . As the unfolding forces of the two higher force steps were close to each other, they could combine into a single large step of ~50 nm. During the following force-decrease scan, we observed two apparent refolding steps at low forces, one at ~5 pN, and another at ~2 pN ( Fig. 2a ). The co-existence of unfolding and refolding steps of same sizes around 5 pN during the stretching process suggests that it corresponds to a near-equilibrium transition operating in this range of forces ( Supplementary Fig. 1c ). We were particularly interested in this transition because its force dependence is close to the range of forces generated by a single myosin motor [53] . If this transition is near-equilibrium in this range of forces it should be largely insensitive to loading rate. To further demonstrate the reversibility of this transition, constant force experiments were carried out in the 4–5 pN range ( Fig. 2c ). Slight increase in force from ~4.1 to ~4.8 pN switched the predominant folded state to the predominant unfolded state. Analysis of the dwell times of each state determined the force-dependent unfolding and refolding transition rates and a critical force of ~4.7 pN ( Supplementary Fig. 1d ). These results confirmed that the ~5 pN transition was insensitive to loading rate in the range tested and reversible around a force of 5 pN, which may be important for physiological myosin-driven conformational switch of α-catenin. Altogether, the highly reproducible force-extension curve we observed characterizes the mechanical response of αC M , and can serve as the basis for further analysis of the force-dependent interaction between αC M and the V D1 domain of the vinculin head. ~5 pN force unfurls αC M exposing the vinculin-binding site To determine whether the αC M near-equilibrium unfolding at ~5 pN corresponds to the unfurling of the VBD domain allowing the stabilization of the V D1 -binding α-helix predicted by structural data [39] , [48] , we performed glutathione S -transferase (GST) pull-down experiments. WT αC M proteins were specifically pulled down with GST-V D1 ( Supplementary Fig. 2a ), as expected from the presence of the VBD domain. To disrupt the V D1 -binding α-helix, we introduced a leucine to proline point mutation in the middle of the α-helix (construct L344P αC M ) [39] . As previously reported [39] , this mutation inhibited the binding of αC M to GST-V D1 ( Supplementary Fig. 2a ). We repeated the force-cycling experiments on L344P αC M . The 5 pN reversible unfolding/refolding step was not observed with the mutant protein ( Fig. 2d and Supplementary Fig. 2b,c ) indicating that the V D1 -binding α-helix was required for proper unfolding/refolding of αC M at ~5 pN. It further suggested that the transition at ~5 pN involves the unfurling of the VBD domain allowing the formation of the vinculin-binding α-helix. We then determined whether αC M mechanical stretching influences V D1 binding. To do so, we counted the number of photobleaching events of Alexa 488-labelled V D1 bound to αC M maintained or not under force. Alexa 488 was conjugated to V D1 following the V D1 labelling protocol used in a previous study of talin-V D1 binding [7] (Methods: ‘Photobleaching counting’). Three typical time trajectories of the fluorescence intensity with zero, one and three photobleaching events, respectively, are presented in Fig. 3a . The number of photobleaching events was very low when no force was applied and increased fivefold when force was increased from 0 to 20 pN ( Fig. 3b , upper panel). Significantly, more tethers showed one photobleaching event at 20 pN force compared with that at 0 pN force. This result is consistent with previous reports suggesting the binding of only one vinculin-binding α-helix per α-catenin central domain [24] . We performed similar experiments with a construct containing three αC M domains. Consistently, using this artificial 3x WT αC M molecule-bearing three potential vinculin-binding sites, we also observed an increase of photobleaching events when forces were increased from 0 to 20 pN, with a number of photobleaching events reaching three at 20 pN ( Fig. 3b ). The rare cases where we observed more than one photobleaching event on WT αC M , or more than three photobleaching events on 3x WT, were likely due to low probability of double or multiple coupling of the Alexa 488 dyes on some V D1 molecules. Altogether these results demonstrate that the mechanical stretching of αC M strongly activates the binding of a single V D1 per VBD domain. 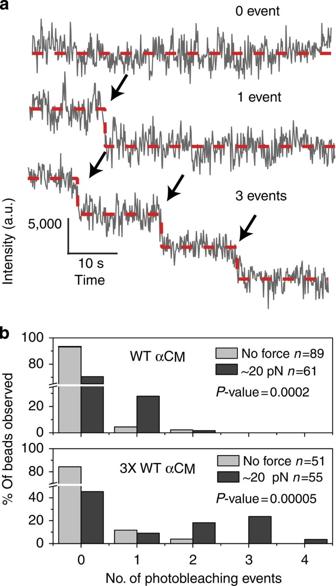Figure 3:Photobleaching counting of VD1bound to WT αCMand 3X WT αCMunder force. (a) Three representative time-lapse traces of the fluorescent intensity measured below individual tethered beads: 0 (WT αCM, no VD1in solution), 1 (WT αCM, VD1in solution) and 3 photobleaching events (3x WT αCM, VD1in solution) were shown for each case. Dashed lines are drawn for visual guidance. (b) Histograms of the percentage of beads with different numbers of photobleaching events observed for WT αCMand 3x WT αCMconstructs. The number of individual tethered beads tested for each condition is denoted by ‘n’ in figure panel. TheP-value was obtained from theχ2test with the null hypothesis that the photobleaching statistics is independent on whether force is applied. Figure 3: Photobleaching counting of V D1 bound to WT αC M and 3X WT αC M under force. ( a ) Three representative time-lapse traces of the fluorescent intensity measured below individual tethered beads: 0 (WT αC M , no V D1 in solution), 1 (WT αC M , V D1 in solution) and 3 photobleaching events (3x WT αC M , V D1 in solution) were shown for each case. Dashed lines are drawn for visual guidance. ( b ) Histograms of the percentage of beads with different numbers of photobleaching events observed for WT αC M and 3x WT αC M constructs. The number of individual tethered beads tested for each condition is denoted by ‘n’ in figure panel. The P -value was obtained from the χ 2 test with the null hypothesis that the photobleaching statistics is independent on whether force is applied. Full size image V D1 binds stretched αC M and inhibits M I domain refolding To correlate the force-dependent binding of V D1 to one of the specific unfolding steps of the αC M molecule described above, we investigated the effect of V D1 on the force responses of αC M . We carried out force cycle experiments in the presence of V D1 in the solution. In a typical force cycle in the presence of 10 nM V D1 , the ~5 pN unfolding step disappeared in the force-increase phase, whereas the two unfolding steps at 10–18 pN remained ( Fig. 4a ). In the force-decrease phase, we observed a small (~2.5 nm) step at ~9 pN, which was not observed in the absence of V D1 , followed by two larger (>15 nm) steps at lower forces also observed in the absence of V D1 . 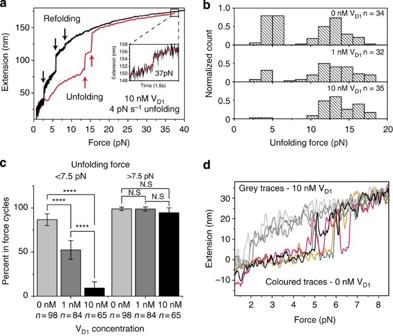Figure 4:Unfolding and refolding of αCMin the presence of VD1. (a) Force-extension curve of αCMin a typical stretch-relax force cycle in the presence of 10 nM VD1. The inset shows a ~3 nm VD1dissociation unfolding step at ~37 pN. (b) Unfolding force histogram obtained from repeating stretch-relax force cycles on a single αCMat different VD1concentrations. (c) Percentages of observed unfolding events at <7.5 pN and >7.5 pN unfolding cycles at different VD1concentrations. The significance indicated by the asterisks is based onP-value calculation from theχ2test with the null hypothesis that the percentages of the unfolding events are independent on the VD1concentration. Four asterisks denote aP-value smaller than 0.0001. The data were collected from eight independent tethers. The error bar denotes 95% confidence interval of probability estimation. (d) Three force-extension curves recorded during three sequential stretch processes between 1 and 9 pN in the presence of 0 nM VD1(coloured traces), where only the ~5 pN unfolding/refolding events occurred. After each stretch, force was jumped to 0.1 pN for 1 min for refolding before the next stretch was performed in the presence of 10 nM VD1(black and grey traces). The ~5 pN unfolding/refolding event was observed during the first stretch cycle (black), but was lost in the subsequent three stretches. Data indare smoothed using 0.05-s time interval. Figure 4: Unfolding and refolding of αC M in the presence of V D1 . ( a ) Force-extension curve of αC M in a typical stretch-relax force cycle in the presence of 10 nM V D1 . The inset shows a ~3 nm V D1 dissociation unfolding step at ~37 pN. ( b ) Unfolding force histogram obtained from repeating stretch-relax force cycles on a single αC M at different V D1 concentrations. ( c ) Percentages of observed unfolding events at <7.5 pN and >7.5 pN unfolding cycles at different V D1 concentrations. The significance indicated by the asterisks is based on P -value calculation from the χ 2 test with the null hypothesis that the percentages of the unfolding events are independent on the V D1 concentration. Four asterisks denote a P -value smaller than 0.0001. The data were collected from eight independent tethers. The error bar denotes 95% confidence interval of probability estimation. ( d ) Three force-extension curves recorded during three sequential stretch processes between 1 and 9 pN in the presence of 0 nM V D1 (coloured traces), where only the ~5 pN unfolding/refolding events occurred. After each stretch, force was jumped to 0.1 pN for 1 min for refolding before the next stretch was performed in the presence of 10 nM V D1 (black and grey traces). The ~5 pN unfolding/refolding event was observed during the first stretch cycle (black), but was lost in the subsequent three stretches. Data in d are smoothed using 0.05-s time interval. Full size image Figure 4b shows unfolding force distributions normalized by the number of force cycles at different V D1 concentrations recorded during force-increase phases on a single tether with more than 30 unfolding events for each condition, which clearly reveals that the frequency of the ~5 pN transition decreases as the V D1 concentration increases. Figure 4c summarizes results from eight different tethers recorded in the absence or in the presence of V D1 at 1 and 10 nM concentrations. The ~5 pN unfolding events were significantly reduced in the presence of 1 nM V D1 , and nearly disappeared in the presence of 10 nM V D1 . Similar results were obtained at higher V D1 concentrations ( Supplementary Fig. 3 ). Interestingly, we found an additional unfolding step at >35 pN associated with a very small step size of ~3.0 nm appearing in the presence of V D1 in solution, which was not observed in the absence of V D1 ( Fig. 4a ). Considering that high forces could favour a transition of the vinculin-binding α-helix from the V D1 -bound state to a V D1 -unbound, extended random coiled peptide chain state, this step could be interpreted as the dissociation of V D1 bound to the vinculin-binding α-helix. Therefore, at a sufficiently high force, V D1 dissociation should occur, accompanied by a small unfolding step during the subsequent helix-to-coil transition of the vinculin-binding α-helix. The ~3 nm unfolding step size observed at ~39 pN was consistent with the estimated extension increase during helix-to-coil transition of the vinculin-binding α-helix at 30–40 pN (Methods: ‘Helix-to-coil transition’). The fact that we observed only one ~3 nm unfolding step at high forces again strongly indicated that a single V D1 -binding helix exists in the αC M construct, which was consistent with our photobleaching experiments ( Fig. 3 ). Similarly, the ~2.5 nm refolding step at ~9 pN that we only observed in the presence of V D1 may be due to the re-binding of V D1 to the unfolded vinculin-binding α-helix of αC M , which induces formation of the α-helix structure of the vinculin-binding site. Consistently, when experiments were performed, at a lower concentration of V D1 (1 nM) to reduce the chance of re-binding during force decrease, we observed that displacement of the bound V D1 at high force could restore the ~5 pN transitions ( Supplementary Fig. 3c ), To investigate whether activation of V D1 binding to αC M requires or not complete unfolding of αC M , we performed force-cycling experiments up to 9 pN at a loading rate of 4 pN s −1 . We selected this maximal force because it only allowed unfolding of the weakest domain at ~5 pN. We found that unfolding the weakest domain was sufficient to activate V D1 binding that abolished the ~5 pN unfolding/refolding events ( Fig. 4d ). The results indicated that unfolding the VBD domain alone was sufficient to activate V D1 binding. Taken together, these results suggested that the vinculin-binding α-helix in αC M could be reversibly exposed by mechanical force of ~5 pN. In addition, they indicated that V D1 binding to the exposed vinculin-binding α-helix inhibited αC M refolding at low force, and that the bound V D1 could be displaced at large forces. V D1 binds to and locks αC M in its open conformation To evaluate to which extent mechanical force increased the affinity of V D1 binding to αC M , we incubated αC M tethers in the presence of 10–100 nM V D1 at low force (1–2 pN) for 10 min before the first stretching. Should V D1 spontaneously bind to the αC M tether at low force during the time, we would expect to observe a loss of the ~5 pN unfolding/refolding step during the first force-increase scan. In three out of four independent experiments, we observed the ~5 pN transition and the two higher force unfolding steps in the first force-increase scan ( Fig. 5a , and Supplementary Fig. 4a,b ), indicating that no V D1 binding had occurred within 10 min incubation at ~2 pN. In addition, we found that the ~5 pN transition was lost in the subsequent force cycles, whereas the two higher force species remained. These results were consistent with V D1 binding occurring after the first stretching procedure, which locked the vinculin-binding α-helix of the M I domain in an open state. In the fourth experiment at 100 nM V D1 , the ~5 pN transition step disappeared in the first force-increase scan, indicating V D1 binding before the force-increase scan. A close examination of the extension time trace revealed that a spontaneous binding of V D1 occurred at ~2 pN at minutes after we introduced V D1 solution, as indicated by an abrupt extension increase ( Fig. 5b ). As V D1 binds to unfolded αC M in seconds under >5 pN forces, these results indicated that mechanical forces above 5 pN strongly promoted V D1 binding to αC M . 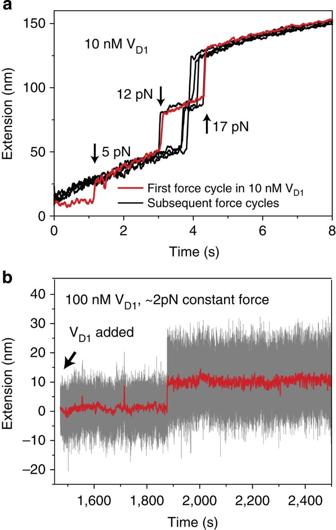Figure 5:Mechanical stretching activates VD1binding to αCM. (a) Extension change of αCMin multiple stretch-relax force cycles in the presence of 10 nM VD1. The VD1solution was slowly introduced at a low force (~1 pN) to avoid αCMunfolding by fluid-drag force. After the VD1solution was introduced, the αCMmolecule was held at ~2 pN for 10 min in the VD1solutions before being stretched for the first time. Data were smoothed with 0.05-s time window. (b) In one out of four experiments after introduction of 100 nM VD1solution at 2 pN, spontaneous binding of VD1occurred indicated by a stepwise unfolding event. For clarity, data are smoothed using 0.5-s time interval. Figure 5: Mechanical stretching activates V D1 binding to αC M . ( a ) Extension change of αC M in multiple stretch-relax force cycles in the presence of 10 nM V D1 . The V D1 solution was slowly introduced at a low force (~1 pN) to avoid αC M unfolding by fluid-drag force. After the V D1 solution was introduced, the αC M molecule was held at ~2 pN for 10 min in the V D1 solutions before being stretched for the first time. Data were smoothed with 0.05-s time window. ( b ) In one out of four experiments after introduction of 100 nM V D1 solution at 2 pN, spontaneous binding of V D1 occurred indicated by a stepwise unfolding event. For clarity, data are smoothed using 0.5-s time interval. Full size image V D1 bound to exposed VBD has a slow off-rate at low force Then, to quantify the stability of V D1 association to mechanically exposed V D1 -binding α-helix under force, we carried out force-jump experiments in which force was alternated between 8 pN to promote rapid V D1 binding, and a high force to dissociate the V D1 from the V D1 -binding α-helix. We found that a single V D1 dissociation event, indicated by a ~3-nm unfolding step, occurred within 10 s after force was switched to ~40 pN ( Fig. 6a ), which was not observed for the L344P mutant ( Fig. 6b ). 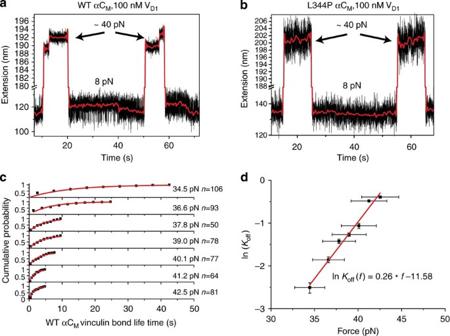Figure 6:High force displaces the bound VD1from the vinculin-binding site in αCM. (a) Extension change of WT αCMduring force jump between ~8 and ~40 pN in the presence of 100 nM VD1. (b) Extension change of L344P αCMduring the same force jump procedure. (c) The histogram of lifetime of VD1bound to αCMat different forces. Red curves are fittings with exponential decay function from which the dissociation rates were obtained. The number of events observed in each condition is denoted by ‘n’ in figure panel. The data were obtained from three individual tethers. (d) The logarithm of the dissociation rate is roughly linearly dependent on force. Red line denotes linear fitting of the log-scaled force-dependent off-rate. From the slope, the transition distance is estimated to be ~1 nm, and the dissociation rate at no force is estimated to be 9.3 × 10−6s−1by extrapolation based on the Bell’s model69.Yerror bars denote 95% confidence interval of off-rate estimation,Xerror bars denote the ~5% relative error of our force calibration method. Figure 6: High force displaces the bound V D1 from the vinculin-binding site in αC M . ( a ) Extension change of WT αC M during force jump between ~8 and ~40 pN in the presence of 100 nM V D1 . ( b ) Extension change of L344P αC M during the same force jump procedure. ( c ) The histogram of lifetime of V D1 bound to αC M at different forces. Red curves are fittings with exponential decay function from which the dissociation rates were obtained. The number of events observed in each condition is denoted by ‘n’ in figure panel. The data were obtained from three individual tethers. ( d ) The logarithm of the dissociation rate is roughly linearly dependent on force. Red line denotes linear fitting of the log-scaled force-dependent off-rate. From the slope, the transition distance is estimated to be ~1 nm, and the dissociation rate at no force is estimated to be 9.3 × 10 −6 s −1 by extrapolation based on the Bell’s model [69] . Y error bars denote 95% confidence interval of off-rate estimation, X error bars denote the ~5% relative error of our force calibration method. Full size image To quantify the force-dependent off-rate of V D1 bound to αC M , we repeated such force-jump for many cycles on native αC M at a variety of forces. The cumulative dissociation time distribution (the percentage of vinculin dissociated at time t ) at various high forces from three independent tethers was obtained ( Fig. 6c ). At each force, the time window of observation was chosen so that in more than 90% of the force-jump cycles vinculin dissociation events were observed. The cumulative dissociation distributions were fitted by an exponential decay function 1−exp(− tK off ), where the parameter K off characterizes the rate of dissociation at force f . We found that the logarithm of K off ( f ) roughly linearly depended on force ( Fig. 6d ), from which the off-rate at low forces could be estimated by linear extrapolation. At <10 pN, the extrapolated off-rate is <10 −5 s −1 . Such an ultraslow dissociation rate of V D1 from exposed V D1 -binding α-helix may explain why the bound V D1 could inhibit refolding of αC M . Altogether, these data indicated a strong stability of the vinculin/α-catenin complex with a rapid formation and slow dissociation in the tension range 5–30 pN. We report here on the mechanical response of the central domain of αE-catenin (αC M ) and its force-dependent binding to the vinculin head (V D1 ), characterized at the single-molecule level, in a physiologically relevant range of forces. Our results show that αC M displays three major unfolding steps, occurring at different forces in the range of 5–20 pN under a physiologically loading rate of 4 pN s −1 . We identified the M I /VBD domain of α-catenin, which contains the V D1 -binding site made of a single α-helix, as the weakest domain that unfolded at ~5 pN. This unfolding step was lost when a single point mutation (L344P) is introduced in the α-helix [39] , as well as when V D1 is bound to αC M . The two larger force-unfolding events are unrelated to binding of V D1 , and are attributed to the unfolding of the sub-domains M II and M III also constituted of helix bundles but not predicted to contain vinculin-binding sites. Structural data suggest that in the folded state, M I /VBD interacts with both M II and M III (ref. 47 ); therefore this interaction may stabilize VBD in its closed conformation, as well as contributing to the stabilization of the M I -M III subdomains. Our results are consistent with a hypothesis that the interaction of the three sub-domains contributes to the stabilization of α-catenin under its close conformation, whereas a moderate 5 pN stretching force disrupt this inter-domain interaction resulting in exposing the vinculin-binding site in the M I /VBD domain. The ~5 pN unfolding and folding transitions are nearly at equilibrium within the loading rates tested in the experiments. These transitions involved a step size of ~16 nm with a critical force of ~4.7 pN at which folding and unfolding are balanced. This transition cannot be explained by the disruption of the inter-domain interactions alone; otherwise much smaller transition steps would be expected as each subdomain has a dimension of only ~3 nm in the folded state. Together with data obtained from L344P mutation and V D1 -binding studies, the ~16 nm step involved in this transition is consistent with a picture that the disruption of the inter-domain interactions at ~5 pN leads to a subsequent unfolding of the M I /VBD α-helix bundle. The extension of an unfolded peptide in random coil and in α-helix conformations is similar, ~17 nm estimated for a chain of extended helices with total ~32 helical turns of 116 residues in the M I domain, and ~15 nm of the same number of residues in the random coil conformation at ~5 pN estimated based on the worm-like chain polymer model with a bending persistence length of ~0.5 nm (reported from 0.4–0.6 nm) [54] , [55] , [56] , [57] . Considering that V D1 -binding occurred at this force range, we reason that the unbundled α-helices in the M I domain at ~5 pN likely assumed a conformation as a chain of extended α-helices rather than a randomly coiled peptide chain. We then demonstrated and characterized in details the kinetics of the force-dependent binding of the V D1 to αC M . Indeed, our results revealed that a characteristic force response of αC M controlled the level of V D1 binding. αC M unfolding at ~5 pN was sufficient to trigger V D1 binding at a nanomolar concentration, which prevented refolding of αC M VBD even after force was released. This binding was observed in the presence of V D1 at concentrations as low as 1 nM and was maximum in the presence of 10 nM V D1 , implying a strong affinity of V D1 to αC M VBD triggered by >5 pN force. Overall, the effect of V D1 binding to the vinculin-binding α-helix in αC M on the characteristic force response of αC M is similar to the leucine to proline mutation at the residue 344 of αC M , both abolishing the ~5 pN unfolding/refolding transitions. These results are also consistent with our observation that V D1 did not bind to L344P αC M in in-vitro pull-down assays. To estimate the increase in the binding affinity of V D1 to αC M by force, we used results from published isothermal titration calorimetry studies, which indicate a K D of 82±19 nM for αC M binding to V D1 at zero force [58] . Based on these calculations, and considering that the apparent V D1 binding to mechanically stretched αC M at ~5 pN was observed at ~1 nM V D1 and maximum at ~10 nM V D1 , we estimated that a force of several piconewton increased the binding affinity of V D1 to αC M by about 100-folds, which may be sufficient to activate auto-inhibited vinculin by competing off its head-to-tail association [59] . Overall, these data provide molecular evidences in strong support of α-catenin as being the force-dependent molecular switch acting at cell–cell junctions to recruit vinculin ( Fig. 7 ), at the basis of the reported tension-dependent growth and adaptation of these junctions [12] , [22] , [26] , [60] . 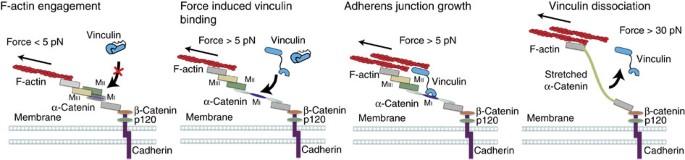Figure 7:Schematics of biphasic dependence of VD1binding to αCMon force. At low force (<5 pN), αCMexists under an auto-inhibited helix bundle conformation that prevents VD1binding. At high force (>30 pN), VD1binding is also inhibited because the α-helix conformation of the vinculin-binding site bound with VD1is unstable. In the intermediate force range (5–30 pN), the auto-inhibited conformation of αCMis released, and the vinculin-binding site is exposed for VD1binding. Figure 7: Schematics of biphasic dependence of V D1 binding to αC M on force. At low force (<5 pN), αC M exists under an auto-inhibited helix bundle conformation that prevents V D1 binding. At high force (>30 pN), V D1 binding is also inhibited because the α-helix conformation of the vinculin-binding site bound with V D1 is unstable. In the intermediate force range (5–30 pN), the auto-inhibited conformation of αC M is released, and the vinculin-binding site is exposed for V D1 binding. Full size image Our results revealed that vinculin head binding is biphasically dependent on force. In the small force range (<5 pN) where αC M existed as natively folded, auto-inhibitory helical bundles, and in the high force range (>30 pN) where the V D1 -binding site was converted from its α-helix conformation to an extended random coiled peptide chain, binding of V D1 was strongly inhibited. Between 5 and 30 pN, binding of V D1 was significantly promoted. As 5 pN is close to the force that can be exerted by a single myosin motor [53] , the low-force regime is likely involved during early adhesion formation with low myosin activity. The high-force V D1 dissociation is also physiologically relevant, as a 30-pN force can be produced by several cooperative myosins or external forces exerted on cells. Ultimately, locking α-catenin in a partially unfolded conformation may regulate cellular adhesion strengthening in a force-dependent manner. Similarly, high forces achieved upon mobilization of multiple myosin molecules pulling on a single αE-catenin molecule via F-actin may eventually release vinculin at >30 pN and then lead to the disruption of the mechanosensitive link [61] . This may explain the disruption of cadherin adhesions observed upon increased cell contraction obtained by increasing RhoA activity [62] . To elucidate these mechanisms, further experiments in cellulo will be required in the future. The force-dependent process centered on α-catenin we unraveled here may further cooperate with the binding of other α-catenin partners to regulate the strength of the cytoskeleton linkage to cell–cell junctions. A ~5 pN force deforms the modulation domain of α-catenin and initializes binding of V D1 . The resulting lockage of α-catenin in a partially unfolded conformation may have a downstream impact on interactions between α-catenin and other junctional and cytoskeleton proteins, such as α-catenin itself, afadin, ZO-1, α-actinin and F-actin. However, further understanding of these processes will require precise structural and biochemical data on these complexes that are lacking so far. Up to date, a complete structural description of αE-catenin under both its closed and open conformations is still lacking. The exact sequential mechanistic pathway by which α-catenin and vinculin bind together at cell–cell contacts has been highly debated within the field. Bakolitsa et al . proposed that αE-catenin VBD binding to vinculin can activate vinculin [58] ; however, previous data suggested that αE-catenin lacking the actin-binding domain, or the VBD domain alone, bound poorly to full-length vinculin in solution unless F-actin is present in the solution [39] , [46] . These results suggested that αE-catenin or the VBD domain alone were not sufficient to activate vinculin by direct interaction with the vinculin head. Nonetheless, as αE-catenin and the VBD domain were not placed under force in those experiments, those results do not rule out the possibility that αE-catenin alone can directly activate vinculin when it is placed under force. Our results demonstrated that V D1 bound to mechanically exposed VBD in αC M under 5–30 pN forces with a nanomolar dissociation constant. This is significantly lower than the K D =~50–90 nM determined for the head-to-tail association of vinculin [59] , [63] . Such a strong affinity between V D1 and mechanically stretched αE-catenin suggests that it may be able to compete off the vinculin head-to-tail association of auto-inhibited vinculin, which warrants future studies. In in vivo conditions, such stably associated activated vinculin may then bind itself to other molecular partners of the junctional complex, such as of F-actin, β-catenin [64] and PtdIns (4,5)P 2 (ref. 58 ), further contributing to the tension-dependent maintenance, strengthening and force-adaptation of cell–cell junctions. To our knowledge, this work provides the first molecular demonstration of a tension-dependent conformational switch for a cadherin-associated protein. It provides a molecular mechanism explaining the local mechanosensitivity of cell–cell junctions, based on tension-dependent unfurling of α-catenin and recruitment of vinculin, a pathway that has been overwhelmingly hypothesized but surprisingly never proven so far. Further studies will be needed to determine whether the pathway is unique at cell–cell junctions or cooperate with similarly operating molecular mechanosensors and/or with more globally distributed mechano-adaptation of the actomyosin cytoskeleton [4] . Together with previous studies on force-dependent binding of vinculin to talin at integrin-mediated cell–matrix adhesions [7] , [8] , this work indicates that tension-dependent unfurling of mechanosensitive proteins and recruitment of actin-binding adaptor proteins to adhesion plaques is a central mode of mechanotransduction at adhesion sites. Further dissection of cell-context modulation of this pathway has broad implications for the understanding of cell adaptation to cell–ECM and cell–cell transduced mechanical load, an important factor of tissue reshaping, tumour progression and collective cell migration. Protein expression and purification A PCR product of the mouse αE-catenin central domain (αC M : residues: 275–735) was cloned into the di-cistronic pDW363 vector, co-expressing the Escherichia coli biotin holoenzyme synthetase (Bir A) [65] . Briefly, the 822–2266 nucleotide fragment of the coding sequence of the mouse αE-catenin cDNA (NM_009818) was amplified by PCR and cloned in phase between the Xho I and Bam HI sites in N-terminal of the lysine-containing sequence recognized by Bir A, replacing the MalE-coding sequence. A 6His-coding sequence followed by a stop codon was added in C-terminal of the αE-catenin sequences. Unique Kpn I and Apa I sites were introduced on both sides of the recombinant αE-catenin, thanks to the following forward: 5′-CTGGTGGCTCGAGCGGTACCGGCGGAGAGCTGGCATACGCT-3′, and reverse: 5′-ATGACCGACTTCACCCGAGGCAAAGGGCCCGGGGCCGGGCATCATCACCATCACCATTGAGGATCCATCATC-3′ primers. We then derived by PCR from this WT Biot-αEcat-6His construct, designated WT αC M throughout this study, a L344P Biot-αEcat-6His named thereafter L334P αC M bearing the L344P point mutation in the VBD domain reported previously to impair vinculin binding [39] . A 3 × WT αC M biotin and 6His-tagged construct, bearing three repeats of the Kpn I- Apa I fragment, was also constructed in the pDW363 vector by combination of PCR amplification and In-Fusion recombination (Clontech). All constructs were validated by full sequencing of the open reading frame. Recombinant Biot-6His fusion proteins were expressed in E. coli BL21 strain and purified using Protino Ni-TED columns (Macherey-Nagel). Protein purity was evaluated by SDS–polyacrylamide gel electrophoresis electrophoresis and protein concentration measured using absorbance at 280 nm. The V D1 (residues: 1–258) construct was expressed as described in previous studies [7] . GST pull-down and western blotting A measure of 10 μg of Biot-αE-cat-6His (WT αC M or L334P αC M ) and 4 μg of GST-V D1 (or GST) were mixed gently with 10 μl of glutathione-sepharose beads in PBS (final volume, 200 μl) for 30 min at room temperature. The beads were washed three times with PBS, then centrifuged for 2 min at 4 °C and incubated in 50 μl of 20 mM reduced glutathione, 50 mM Tris-HCl buffer pH 8 for 10 min at room temperature. GST-V D1 (or GST) with associated αE-catenin were recovered in the supernatant after centrifugation. Proteins were resolved on 10% polyacrylamide gels (Invitrogen) by conventional SDS–polyacrylamide gel electrophoresis and Coomassie blue staining. Single-molecule manipulation The single-molecule α-catenin pulling experiments were done on a home-made high-force magnetic tweezers setup with laminar flow channels with a NTA-Cu 2+ functionalized coverslip for specific immobilization of αC M . The force calibration was done for each individual tethered bead measured in experiments, which had an ~5% relative error. The details of the design and control of the magnetic tweezers setup were published previously [49] . Protocols of coverslip functionalization, sample preparation, single-protein stretching experiments and force calibration have been published in our previous studies of Filamin A protein [50] , [51] . Briefly, the channels were prepared by the following procedure: 20 × 32 mm 2 1.5# coverslips were cleaned by ultrasonication in detergent, acetone and isopropanol for 30 min each, followed by 15 min of oxygen plasma treatment. The cleaned coverslips were silanized by incubation in 1% APTES (Sigma) in methanol for 20 min, rinsed thoroughly with methanol and cured for 20 min in oven at 110 °C. A laminar flow channel was made by sandwiching the silanized coverslip and a 20 × 20 mm 2 clean non-functionalized coverslip with two parallel stripes of double-sided tape as spacer. The laminar flow channel was further treated by 0.5% glutaraldehyde for 1 h followed by incubation with 3 μm diameter amine-coated polysterene beads (polysciences) for 20 min and then with 10 μg ml −1 NH2-NTA for 6 h. The channel was then treated with 500 mM Tris pH 7.4 for 20 min and 0.04% (w/v) CuSO 4 for 10 min. The Cu 2+ charged channels were then blocked in PBS, 1% BSA, 0.0002% Tween-20 overnight before stretching experiment. 6His and biotin double-tagged αC M molecule (0.002 mg ml −1 ) were introduced in the channel and incubated for 20 min before introduction of 2.8 μm diameter streptavidin-coated paramagnetic beads (M270 streptavidin, Dynabeads) to form tethers. A syringe pump was used for slow buffer exchange (~5 μl min −1 ). The drag force applied to αC M during buffer exchange was estimated to be less than 1 pN. The pulling experiments were done in 40 mM phosphate buffer pH 7.4, 300 mM NaCl, 5 mM β-mercaptoethanol and 10 mg ml −1 BSA at 22 °C with various V D1 concentrations. Raw extension data were recorded at a sampling rate of 200 Hz. In Figs 2b,d , 4a,d and 5a,b , those are smoothed using the fast Fourier transform (FFT)-smooth function of OriginPro 9.0 in order to improve the clarity of data representation. The unfolding steps of the molecule were detected using an in-house written Matlab programme. Briefly, a delta-function was calculated from the raw time lapse data. Candidate unfolding step positions were picked by peaks in the delta-function with height above a threshold of 10 nm. To determine the unfolding step size, the data points across the individual steps were fitted to a Heaviside step function with an additional linear term that take into account the continuous extension increase because of force change in the force scans. Finally, a t -test was carried out to test the height difference before and after the individual identified steps. Only statistically significant ( P -value<0.01) steps were considered. Force calibrations methods The force applied to a bead depends on both the magnets–bead distance and the maximal magnetization of the bead. The latter is determined by the number of nano-magnetites in the bead, which has a large variation from one bead to another. At a fixed magnets–bead distance, this results in a large variation in force. According to our previous studies, forces applied to the weakest and the strongest M280 dynabeads at the same magnets–bead distance can differ by 100% (ref. 49 ). In the single-protein manipulation studies of unfolding and refolding of αC M molecules, force was calibrated for individual beads based on their thermal fluctuations under force. A small relative error in force calibration (~5%) was ensured, which was mainly caused by the variation in the size of beads [49] . In the photobleaching assay, a fixed magnets–bead distance was maintained and the sample chamber was scanned over 1 h time scale such that tethers in the chamber were subjected to the force as homogeneous as possible. Then, photobleaching assay was performed. As in this assay, the thermal motions of the beads were not tracked, the force estimated represented the average force and therefore had a significantly larger error compared with the single-molecule manipulation assay. To ensure most beads were subject to large enough force to unfold the αC M molecules, a fixed magnets–bead distance was chosen to have a relatively large average value of 20 pN. Photobleaching counting The photobleaching counting of the number of Alexa 488-labelled V D1 bound to a single WT αC M or 3X αC M under force were carried out using a total internal reflection microscope similar to the one described in the previous study of talin–vinculin interactions [7] . Force estimated in the photobleaching assay represented the average force and therefore has a significantly larger error compared with the single-molecule manipulation assay. Labelling and purification of the V D1 with Alexa 488 dye were based on the commercial microscale protein labelling kit (A30006) following the manufacturer’s protocol. The Alexa Fluro-488 reactive dye has a tetrafluorophenyl ester, which reacts efficiently with primary amines of proteins to form stable dye–protein conjugates. The solution containing 50 μg ml −1 labelled V D1 was added to the flow-chamber coated with WT αC M or WT 3X αC M constructs. These constructs were subjected to force and incubated for 1 h, then unbound V D1 was flushed away before counting the number of bound V D1 by photobleaching events similar to previous studies of talin–vinculin interaction. The images of TIRF fluorescence at 488 nm were taken for 1 min using Olympus IX71 (TIRF) microscope with a 1.45 numerical aperture, × 100 objective. Images were further analysed using in-house written Igor programme. Briefly, a region of interest containing a tethered magnetic bead was chosen and the total fluorescence intensity of this region of interest was recorded. The auto-fluorescence of the magnetic beads contributed to a background intensity, which was stable at our experimental time (~60 s) without any abrupt changes. For a tether with bound labelled V D1 , photobleaching of single-dye molecules showed an abruptly decrease in fluorescence intensity, which allowed us to count the number of labelled V D1 associated to the tether. Single-dye photobleaching events were identified following the method developed by del Rio et al . in their paper on force-dependent vinculin binding to talin [7] . Spontaneous stepwise decreases of fluorescent intensity in the time trajectories of the total fluorescence underneath the magnetic beads were identified as photobleaching steps of Alexa 488-labelled V D1 . These photobleaching steps were not present in control experiments when Alexa 488-labelled V D1 was not added. In that case, only smooth exponential decay of auto-fluorescence of the bead was observed. The number of tethered beads tested for the WT αC M at no force and 20 pN of applied force was 89 and 61, respectively. For the WT 3X αC M , the total number of tethered beads tested was 51 and 55 for no force and 20 pN force, respectively. Determination of transition rates at constant forces The force-dependent kinetic rates of the near-equilibrium unfolding/refolding transitions between 4 and 6 pN were obtained by fitting constant force extension fluctuation time traces to a Modified Hidden Markov model. An in-house written Matlab programme based on the Viterbi algorithm was used to find emission distribution and corresponding folded/unfolded state sequence with maximum likelihood [66] . The lifetime distributions of each state were then fitted to an exponential distribution to obtain their characteristic lifetime t . The unfolding and refolding transition rates at a given force were calculated as the inverse of the fitted characteristic lifetime of the unfolded and folded states. The distance to the transition state was calculated by the slope of the linear fit of the natural logarithm of the unfolding and refolding rates at different forces as described previously [67] . Helix-to-coil transition estimation Crystal structures were available for vinculin head binding to the V D1 -binding α-helix of αE-catenin such as 4EHP. V D1 can only bind to the VBD of αE-catenin if the V D1 -binding domain is under α-helix conformation. When interacting with V D1 , the vinculin-binding site of αE−catenin adopts an α-helical structure with six turns of alpha helix that consists of around 22 residues and span a length of around 3.2 nm (0.54 nm per turn). Although at 25–40 pN, the length of a random coil of 22 amino acids is predicted to be 6.1–6.7 nm based on the worm-like-chain polymer model [68] with a persistent length of 0.5 nm estimated from previous protein unfolding experiments [56] (0.4–0.6 nm). Therefore, the size of steps expected for the helix-to-coil transition of the vinculin-binding α-helices when the vinculin head domain dissociates is ~2.9–3.5 nm. How to cite this article: Yao, M. et al . Force-dependent conformational switch of α-catenin controls vinculin binding. Nat. Commun. 5:4525 doi: 10.1038/ncomms5525 (2014).